Critical fictive temperature for plasticity in metallic glasses A long-sought goal in metallic glasses is to impart ductility without conceding their strength and elastic limit. The rational design of tough metallic glasses, however, remains challenging because of the inability of existing theories to capture the correlation between plasticity, composition and processing for a wide range of glass-forming alloys. Here we propose a phenomenological criterion based on a critical fictive temperature, T fc , which can rationalize the effect of composition, cooling rate and annealing on room-temperature plasticity of metallic glasses. Such criterion helps in understanding the widespread mechanical behaviour of metallic glasses and reveals alloy-specific preparation conditions to circumvent brittleness. Despite their similar inherent amorphous structure, which endows metallic glasses with high strength and elasticity [1] , [2] , [3] , [4] , they exhibit a broad range of damage tolerance, from ideal brittle to remarkably tough [5] , [6] , [7] , [8] . Such wide spectrum of mechanical properties is in stark contrast to oxide glasses, and understanding the origin has been the focus of the metallic glass community for the last decade [6] , [7] , [8] , [9] , [10] , [11] , [12] . Mechanical response of a metallic glass is further influenced by extrinsic effects, such as cooling rate [13] , sample size [14] , [15] and testing conditions (temperature and strain rate) [16] , [17] . Besides these extrinsic factors, the understanding of composition-dependent plasticity in metallic glasses continues to defy proposed theories. For example, Pd-based metallic glass is significantly more brittle compared with Pt-based metallic glass prepared at a similar cooling rate [18] . Plasticity of Zr-Cu-Al metallic glasses is very sensitive to composition, whereas their microstructure and elastic constants are largely unaffected [19] , [20] . The atomic-level structure underlying this different mechanical response of metallic glasses is difficult to characterize. Computational modelling offers some insight about the composition–structure–property relationship; however, the lowest achievable cooling rates in simulation are still several orders of magnitude higher than experimental cooling rates [11] . Following the analogy from crystalline metals, the toughness of metallic glasses has been correlated with their elastic constants [6] , [9] , [21] , [22] . Higher Poisson’s ratio or lower G / B ( G : shear modulus, B : bulk modulus) ratio is predicted to result in higher toughness in metallic glasses, mechanistically by increasing the resistance for crack opening compared with shear band formation and extension. Therefore, a high Poisson’s ratio or low G / B has been often used as an indicator for designing tough metallic glasses [6] , [9] . In recent years, increasing experimental evidence has mounted about the limited applicability of G / B in predicting the mechanical response of metallic glasses [18] , [23] , [24] , [25] . In particular, a marginal change in elastic constants cannot account for the sever annealing-induced embrittlement observed in metallic glasses [23] . These findings suggest that a simple, elastic moduli-based approach does not capture the essential features of the multifaceted plasticity problem in amorphous metals. A comprehensive description for the mechanical behaviour of metallic glasses requires the understanding of the complex interplay between their composition, processing, structure and properties. In polymer and oxide glasses, it has been widely observed that the properties of a glass at room temperature are reminiscent of its supercooled liquid at the fictive temperature ( T f ) [26] , [27] , [28] . For metallic glasses, it has been shown that the room-temperature elastic constants can be directly correlated with the values of the supercooled liquid through the linear Debye-Grüneisen thermal expansion [29] . Therefore, knowledge of the supercooled liquid state and the fictive temperature can provide a key insight about the room-temperature properties of metallic glasses. In this work, we study the effect of fictive temperature on the room-temperature plasticity of bulk metallic glasses (BMGs). Samples that are brittle at room temperature may deform plastically at higher temperatures as reported earlier [17] . However, the goal of the present study is to understand the room-temperature mechanical response and its correlation with the properties of their supercooled liquids among different glass-forming alloys. Three BMG formers are considered: Pt 57.5 Cu 14.7 Ni 5.3 P 22.5 (Pt-BMG), Pd 43 Cu 27 Ni 10 P 20 (Pd-BMG) and Zr 44 Ti 11 Cu 10 Ni 10 Be 25 (Zr-BMG). In this study, 2.5% strain to failure is set as the ductile – brittle transition to accommodate ±0.5% measurement error, because even the most brittle metallic glasses still exhibit approximately 2% elastic strain [4] . Our results show that the room-temperature plasticity of BMGs decreases with lowering the fictive temperature, and falls below the ductile–brittle transition at a critical fictive temperature, T fc , which is characteristic of the BMG former. We demonstrate that T fc is a key parameter that defines the mechanical behaviour of BMGs and its sensitivity to cooling rate and annealing. Bending strain and elastic constants Room-temperature strain to failure corresponding to different fictive temperatures for the considered BMG formers is shown in Fig. 1a . 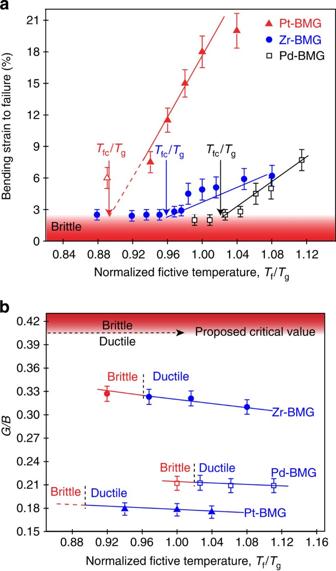Figure 1: Effect of fictive temperature on strain and elastic constants. (a) Room-temperature bending strain to failure as a function of normalized fictive temperature for Pt-BMG, Zr-BMG and Pd-BMG. The critical fictive temperature for ductile–brittle transition is 0.89Tg, 0.96Tgand 1.02Tgfor Pt-BMG, Zr-BMG and Pd-BMG, respectively. The open triangle is the strain to failure for Pt-BMG annealed at 0.89Tgfor 30 days. (b)G/Bratio shows a weak dependence on fictive temperature. TheG/Bratio for the embrittled BMGs is well below the proposed critical value for ductile–brittle transition. The temperature scale is normalized to the calorimetric glass transition temperature, T g , listed in Table 1 . A common feature of all three BMGs is that their strain to failure decreases with lowering T f and it drops below the ductile – brittle transition for T f < T fc . The plastic strain appears to correlate with T f − T fc , which is remarkably similar to the temperature dependence of free volume ( v f ~ T − T 0 , v f is free volume and T 0 is Vogel–Fulcher–Tammann temperature) predicted by the Vogel–Fulcher–Tammann equation [30] . Besides this common trend, there are several notable distinctions among three BMGs. The strain to failure for the Pt-BMG remains significantly higher than that for the Zr-BMG and the Pd-BMG after annealing at the same normalized fictive temperatures. The T fc for the Pd-BMG former is highest among considered BMG formers and occurs above calorimetric T g , whereas for the Zr-BMG former and the Pt-BMG this transition is below T g . Figure 1b shows the variation in G / B values as a function of normalized fictive temperature. The G/B values for the as-quenched BMGs are listed in Table 1 . The change in G/B with fictive temperature is small even though plasticity changes significantly. For all three BMG formers, the G/B ratio corresponding to the critical fictive temperature T fc is far below that of the previously proposed lower limit of 0.41 for brittleness [9] . Figure 1: Effect of fictive temperature on strain and elastic constants. ( a ) Room-temperature bending strain to failure as a function of normalized fictive temperature for Pt-BMG, Zr-BMG and Pd-BMG. The critical fictive temperature for ductile–brittle transition is 0.89 T g , 0.96 T g and 1.02 T g for Pt-BMG, Zr-BMG and Pd-BMG, respectively. The open triangle is the strain to failure for Pt-BMG annealed at 0.89 T g for 30 days. ( b ) G / B ratio shows a weak dependence on fictive temperature. The G / B ratio for the embrittled BMGs is well below the proposed critical value for ductile–brittle transition. Full size image Table 1 Calorimetric T g measured at a heating rate of 20 K min −1 , T fc , T g − T fc and G / B ratio for the considered BMG formers. Full size table Thermal embrittlement of metallic glasses, as displayed in Fig. 1a , is typically attributed to reduction in free volume through structural relaxation [31] , [32] . The structural relaxation time at T g is approximately 100 s and increases exponentially with decreasing temperature [33] . At temperature far below T g , it is impractical to attain completely relaxed glassy state. This suggests that a metallic glass exhibiting T fc far below T g should not become brittle during experimental annealing time. To test this correlation, Pt-BMG was annealed for 30 days at its estimated T fc of 446 K, which is 57 K below the T g . The sample remained ductile and displayed a bending strain of 6% (open triangle in Fig. 1a ). According to the relaxation kinetics, it would take about 30 years to structurally relax Pt-BMG at 446 K (ref. 34 ). In contrast, the Zr-BMG with a T fc of only 25 K below its T g , is sensitive to embrittlement during annealing near T g (ref. 23 ). The Pd-BMG is even more susceptible to annealing-induced embrittlement because of its T fc above T g , which corresponds to a relaxation time of only 50 s. Consequently, the difference between T g and T fc of a metallic glass correlates with its resistance to annealing-induced embrittlement. Effect of cooling rate Mechanical properties of some BMGs strongly depend on the cooling rate during vitrification, whereas others show little or no variation [13] , [18] , [21] . The degree of cooling-rate sensitivity among BMG formers can be rationalized based on their T fc values. If the cooling rate is sufficiently fast, the resulting T f is higher than T fc , and the BMG is ductile. A slower cooling rate will result in lower T f , and the glassy state will become brittle if T f drops below T fc . Typical cooling rates that result in bulk metallic glass formation (thickness >1 mm) span over four orders of magnitude ranging from 0.1 to 1,000 K s −1 (ref. 35 ). Experimental measurements in a wide range of glass-forming liquids reveal that T f decreases by 5–10 K for every order-of-magnitude decrease in cooling rate [28] , [36] , [37] . The maximum variation in T f , as a result of cooling rate, can be approximated to 40 K for BMG formers ( Fig. 2 ). This implies that for a BMG whose T fc differs from its T f by more than 40 K, its ductile or brittle behaviour will remain essentially unaffected by the cooling rate. BMG formers with T f − T fc >40 K will be ductile and the ones with T f − T fc ≤40 K will be brittle for typical cooling rates used in BMG formation. In contrast, the BMG formers with T fc in the proximity of T f ( Fig. 2 ) will be sensitive to the cooling rates. 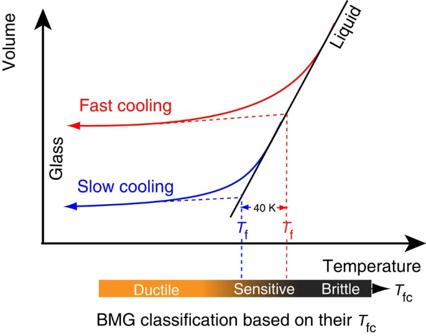Figure 2: The predicted mechanical behaviour of BMG formers under typical cooling rates. The maximum variation inTfis about 40 K as a result of critical cooling rate, which spans over four orders of magnitude among BMG formers. BMG formers withTfcout of the accessibleTfrange are either always ductile (Tf−Tfc>40 K) or brittle (Tf−Tfc≤40 K). However, BMG formers withTfc~Tfcan change from ductile–brittle within practical cooling-rate variations. Figure 2: The predicted mechanical behaviour of BMG formers under typical cooling rates. The maximum variation in T f is about 40 K as a result of critical cooling rate, which spans over four orders of magnitude among BMG formers. BMG formers with T fc out of the accessible T f range are either always ductile ( T f − T fc >40 K) or brittle ( T f − T fc ≤40 K). However, BMG formers with T fc ~ T f can change from ductile–brittle within practical cooling-rate variations. Full size image Isothermal embrittlement diagrams The existence of T fc is experimentally manifested in the cooling-rate-dependent mechanical behaviour of BMGs. Several BMGs such as Fe-based and Mg-based, which are known to be typically brittle, become ductile when cooled at higher rates [21] , [38] . The cooling rate ( R e ) to prevent embrittlement and its relation with the T fc can be understood from isothermal time–temperature–transformation (TTT) diagrams for embrittlement ( Fig. 3 ). The embrittlement time is the annealing time required to decrease the bending strain below the ductile – brittle limit. The embrittlement time decreases with increasing temperature till T fc and then increases abruptly before decreasing again with further increase in temperature. The discontinuity at T fc is related to the change in embrittlement mechanism from structural relaxation ( T ≤ T fc ) to crystallization ( T > T fc ). The T fc is the highest temperature at which a metallic glass can embrittle by structural relaxation. Consequently, the embrittlement of a glassy state through relaxation is fastest at T fc that corresponds to the ‘nose’ of embrittlement curves in Fig. 3 . The embrittlement time at the nose, t e , determines the cooling rate R e to vitrify a ductile glassy state. The t e values for Pd-BMG, Zr-BMG and Pt-BMG are 50 s, 5,000 s, and 9E–9 s, respectively. These values scale with the difference T g − T fc (Pt-BMG>Zr-BMG>Pd-BMG). The short t e indicates that R e is highest for Pd-BMG among the considered BMG formers. The critical cooling rate ( R c ) for glass formation, however, follows the opposite trend and is lowest (0.09 K s −1 ) for the Pd-BMG [35] . This suggests that the critical cooling rates for avoiding crystallization and embrittlement are not directly correlated. 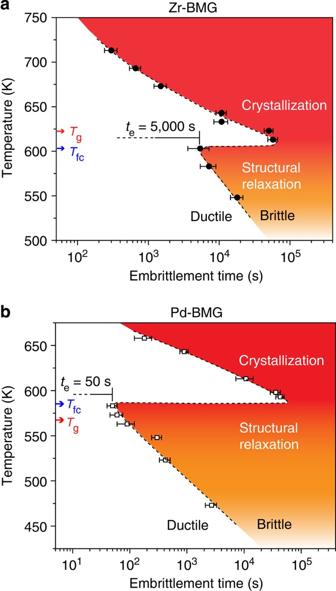Figure 3: TTT diagrams for embrittlement. TheTfcis the highest temperature where embrittlement can occur owing to structural relaxation. AboveTfc, the embrittlement time increases abruptly because of change in origin of embrittlement from structural relaxation to crystallization. The time (te) atTfcdefines the nose of TTT diagrams for embrittlement. The measuredteis 5,000 s for Zr-BMG (a) and 50 s for Pd-BMG (b). Figure 3: TTT diagrams for embrittlement. The T fc is the highest temperature where embrittlement can occur owing to structural relaxation. Above T fc , the embrittlement time increases abruptly because of change in origin of embrittlement from structural relaxation to crystallization. The time ( t e ) at T fc defines the nose of TTT diagrams for embrittlement. The measured t e is 5,000 s for Zr-BMG ( a ) and 50 s for Pd-BMG ( b ). Full size image A comprehensive framework to account for the diverse mechanical behaviour of metallic glasses can be constructed based on the knowledge of T f − T fc . According to this criterion, all metallic glasses can be broadly classified into two groups: T f − T fc <0 (type I) and T f − T fc >0 (type II). For type I metallic glasses, the embrittlement nose time is shorter than the crystallization nose time and, consequently, the critical cooling rate to prevent embrittlement is higher than the critical cooling rate for glass formation ( Fig. 4a ). Here T f is the fictive temperature of a glass vitrified at its critical cooling rate for glass formation. The magnitude of T f − T fc determines their mechanical behaviour and its sensitivity to cooling rate and annealing. Metallic glasses with a small negative T f − T fc are sensitive to preparation conditions and can change from ductile to brittle or vice versa with varying cooling rates. For metallic glasses with large negative T f − T fc , the embrittlement nose time is much shorter than the crystallization nose time. Consequently, their bulk states are always brittle. This explains why Fe-based and Mg-based metallic glasses require high cooling rates, unachievable in bulk form, to vitrify into a ductile state [21] . 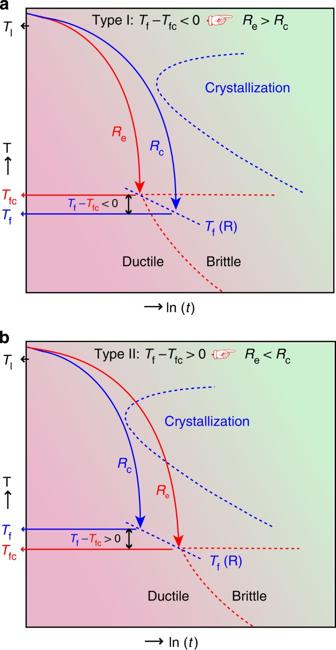Figure 4: Classification of BMG formers based onTf−Tfcvalues. (a) Type I metallic glasses (Tf−Tfc<0) exhibit an embrittlement nose time shorter than the crystallization nose. As a result, these BMG formers are typically brittle but can be made ductile if a cooling rate higher thanReis applied. (b) For type II metallic glasses (Tf−Tfc>0), the embrittlement nose time is longer than the crystallization nose time; therefore, these BMG formers are always ductile. In both cases, variation ofTfwith cooling rate is shown. For practical convenience, calorimetricTgcan be used to approximateTf. Figure 4: Classification of BMG formers based on T f − T fc values. ( a ) Type I metallic glasses ( T f − T fc <0) exhibit an embrittlement nose time shorter than the crystallization nose. As a result, these BMG formers are typically brittle but can be made ductile if a cooling rate higher than R e is applied. ( b ) For type II metallic glasses ( T f − T fc >0), the embrittlement nose time is longer than the crystallization nose time; therefore, these BMG formers are always ductile. In both cases, variation of T f with cooling rate is shown. For practical convenience, calorimetric T g can be used to approximate T f . Full size image Type II metallic glasses ( T f − T fc >0) exhibit an embrittlement nose time that is longer than the crystallization nose time ( Fig. 4b ). Hence, their critical cooling rate for embrittlement is lower than the critical cooling rate for glass formation. These metallic glasses are always ductile in the as-cast bulk state and the magnitude of T f − T fc indicates their resistance to annealing-induced embrittlement. Metallic glasses with a large positive T f − T fc (for example, Pt-BMG) do not become brittle under practical annealing conditions, because their embrittlement time (≈relaxation time) at T fc is extremely long. In contrast, metallic glasses with a small positive T f − T fc (for example, Zr-BMG) are ductile in the as-cast state but are susceptible to annealing-induced embrittlement because of their fast relaxation at T fc . According to this critical fictive temperature viewpoint, the knowledge of T fc and T f is sufficient to understand a BMG’s resistance to annealing-induced embrittlement, cooling rate sensitivity and critical cooling rate for plasticity. In practice, T f measured by method of integration from differential scanning calorimeter (DSC) heating curves is typically few degrees lower than the T g (ref. 39 ). Therefore, calorimetric T g values can be used as a good approximation of T f for the practical application of plasticity criteria outlined here. Our experimental results validate the use of calorimetric T g for prediction of mechanical response of BMG formers. Pt-BMG with T g − T fc ~57 K is ductile at any cooling rate and exhibits higher resistance to annealing embrittlement. Zr-BMG with T g − T fc ~25 K is ductile in the as-cast state, but becomes brittle during sub- T g annealing [23] . Pd-BMG with T g − T fc ~−12 K changes from ductile to brittle when the cooling rate is decreased below 50 K s −1 (ref. 18 ). The absolute values of T fc and hence T g − T fc are a function of sample size because of the size-dependent plasticity of BMGs [13] , [15] . 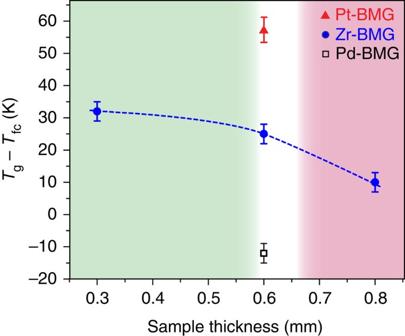Figure 5: Effect of sample size on the critical fictive temperature. Tg−Tfcvalues for Zr-BMG of different thicknesses are compared with that of 0.6-mm thick Pt-BMG and Pd-BMG samples. The results demonstrate that the effect of alloy composition is more pronounced than sample size. Therefore,Tfcmeasured for any sample size can be used in theTg−Tfccriterion for plasticity. Figure 5 shows T g − T fc for Zr-BMG samples of different thicknesses. T g − T fc increases with decreasing temperature. However, this size dependence is much smaller than the effect of composition on T g − T fc . For Pt-BMG of 0.6 mm thickness, the T g − T fc is larger than that of the 0.3-mm thick Zr-BMG. Similarly, the T g − T fc of 0.8-mm thick Zr-BMG is larger than that of the 0.6-mm thick Pd-BMG. Thus, T g − T fc values measured for any sample size allow to predict the mechanical behaviour of different glass-forming alloys. Figure 5: Effect of sample size on the critical fictive temperature. T g − T fc values for Zr-BMG of different thicknesses are compared with that of 0.6-mm thick Pt-BMG and Pd-BMG samples. The results demonstrate that the effect of alloy composition is more pronounced than sample size. Therefore, T fc measured for any sample size can be used in the T g − T fc criterion for plasticity. Full size image In summary, we propose T g − T fc criterion to predict the room-temperature mechanical behaviour and its sensitivity to cooling rate and annealing-induced embrittlement for metallic glasses. We envision that application of structural models [40] , [41] can reveal the microscopic origin of such a critical fictive temperature to design tough metallic glasses. Sample preparation Pt 57.5 Cu 14.7 Ni 5.3 P 22.5 and Pd 43 Cu 27 Ni 10 P 20 alloys were prepared by induction melting the constituents in vacuum-sealed quartz tube. The alloys were subsequently fluxed with B 2 O 3 at 1,000 °C for 600 s. The fluxed alloys were re-melted and water-quenched in 3-mm diameter quartz tubes to prepare the bulk amorphous samples. Amorphous Zr 44 Ti 11 Cu 10 Ni 10 Be 25 was acquired from Liquidmetal Technologies. Rectangular beams of 0.6±0.05 mm thickness were machined from the bulk amorphous samples. To achieve the desired T f , the beams were annealed at various temperatures (annealing temperature= T f ). Annealing times were chosen two times longer than the relaxation time, to ensure that the equilibrium had been reached at T f . Crystallization can be ruled out, because the annealing times are at least an order of magnitude shorter than the crystallization times. After annealing, the samples were water-quenched to obtain the glassy state corresponding to different fictive temperatures. Characterization The samples were characterized thermally by DSC and structurally by X-ray diffraction. The glass transition temperature, T g , was measured from DSC heating curves recorded at a heating with 20 K min −1 . Elastic constants were calculated from the shear and longitudinal sound velocities measured at room temperature by an ultrasonic technique. The bending strain to failure was measured by bending the beams around mandrels of different radii at room temperature [14] . The samples were mirror polished before the bending tests. The bending strain corresponds to t /2 r ( t is the thickness of the samples and r is the radius of the mandrel). The average bending strain and error bars were calculated by testing five samples for each fictive temperature. Construction of TTT diagrams for embrittlement The samples were isothermally annealed at various temperatures followed by water quenching to room temperature. The embrittlement time corresponds to the annealing time for which the room-temperature bending strain to failure reduces to 2.5% or lower. TTT diagrams for embrittlement were constructed by plotting the log of isothermal embrittlement times as a function of temperature. How to cite this article: Kumar, G. et al. Critical fictive temperature for plasticity in metallic glasses. Nat. Commun. 4:1536 doi: 10.1038/ncomms2546 (2013).